Experimental demonstration of graph-state quantum secret sharing Quantum communication and computing offer many new opportunities for information processing in a connected world. Networks using quantum resources with tailor-made entanglement structures have been proposed for a variety of tasks, including distributing, sharing and processing information. Recently, a class of states known as graph states has emerged, providing versatile quantum resources for such networking tasks. Here we report an experimental demonstration of graph state-based quantum secret sharing—an important primitive for a quantum network with applications ranging from secure money transfer to multiparty quantum computation. We use an all-optical setup, encoding quantum information into photons representing a five-qubit graph state. We find that one can reliably encode, distribute and share quantum information amongst four parties, with various access structures based on the complex connectivity of the graph. Our results show that graph states are a promising approach for realising sophisticated multi-layered communication protocols in quantum networks. The potential benefits of using quantum mechanics to carry out information processing in a connected world are now well established [3] . While the algorithmic speedups offered by quantum computers [4] and the robust security provided by quantum key distribution [5] are outstanding improvements over what is classically achievable, in recent years many new protocols have emerged in the setting of quantum networks. These protocols include quantum coin flipping [6] , [7] , [8] , [9] , blind quantum computation [10] , [11] and distributed and secure quantum computation [12] , [13] . One of the most useful protocols for distributed quantum information processing is quantum secret sharing [14] , [15] . In this protocol, one player is able to distribute a secret (classical or quantum information) to a network of players, such that only authorized sets of players can access the secret and unauthorized sets obtain no information. Secret sharing has many useful applications in network-based scenarios, such as auctioning, remote voting, secure money transfer and multiparty secure computation. The first classical protocols for secret sharing of information, in the form of a bit string, were introduced in 1979 by Shamir [16] and Blakely [17] , with quantum versions later developed [14] , [15] for sharing classical and quantum secrets using quantum bits, or qubits. Most recently, secret sharing protocols have been unified under the framework of graph states [18] , [19] , [20] —highly nonlocal quantum resources made from a network of entangled qubits that can be used to share both classical and quantum secrets. One of the most promising features of graph state-based quantum secret sharing is the natural capacity of the entangled resource states to be integrated into more complex networking protocols and their entanglement exploited for extended functionality [21] , [22] , [23] . Indeed, graph states are also the basis for universal measurement-based quantum computation [24] , [25] , [26] , [27] , [28] , [29] , error correction [30] , [31] , [32] , [33] , [34] , [35] , [36] , [37] and blind quantum computation [10] , [11] , making them versatile resources for distributed quantum information processing. In this work, we report an experimental demonstration of graph state-based secret sharing of classical and quantum information using photons in a linear optics setup. We first show how a five-qubit graph state can be used for sharing a classical secret amongst four players using quantum channels (CQ)—secure against a distrusted channel between the dealer (the party that shares the secret) and the four players. We then show how the same five-qubit graph state can be used to share a quantum secret with quantum channels (QQ). Finally, we demonstrate secret sharing of quantum information which is verified as secure against distrusted channels between the dealer and the other players (SQQ). This is achieved by combining classical Shamir–Blakely protocols [16] , [17] with CQ and schemes for sharing quantum secrets recently introduced in refs 16 , 17 , 36 . With our results we therefore demonstrate the practical potential of graph state quantum secret sharing, as well as the capacity for integrating several cryptographic protocols in this setting. The results and their analysis show some of the key advantages of using graph states for quantum communication protocols in future quantum networks. Resource characterization The setup used to demonstrate graph-state quantum secret sharing is shown in Fig. 1a and generates the five-qubit graph state shown in Fig. 1b , which acted as a resource state for carrying out the protocols. In the graph state, there is an initial entanglement between the dealer’s qubit (centre qubit) and that of each of the four players (the outer qubits). The state was generated using the method described in ref. 35 , where a birefringent photonic crystal fibre (PCF) generates a polarization-entangled pair of photons in the state , with H and V referring to horizontal and vertical polarization. The entangled photons are generated at non-degenerate signal and idler wavelengths of 625 and 860 nm. A second PCF generates heralded single photons at the signal wavelength (see Methods). Both PCF sources were pumped by the same pulsed laser. The signal photons from the two PCF sources were then overlapped at a polarizing beamsplitter (PBS) to perform a postselected fusion operation [39] , leaving a three-photon entangled GHZ state . This state can be converted by local operations to a linear graph state , where the single-qubit computational basis states |0 and |1 are encoded as horizontal and vertical polarizations, and therefore are encoded as diagonal and antidiagonal plane polarizations. These 45° rotations are applied to the two signal photons emerging from the PBS fusion operation using half-wave plates (HWPs). 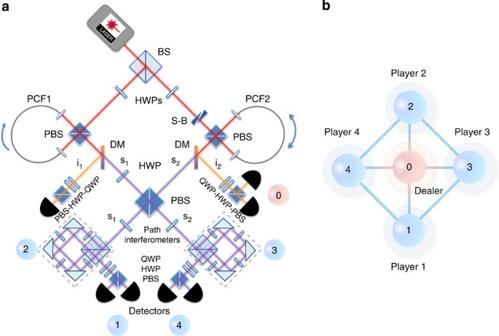Figure 1: Experimental setup. (a) Setup used to generate the graph state resource for secret sharing. Two photonic crystal fibre (PCF) sources are pumped using a Ti:Sapphire laser producing picosecond pulses at 724 nm. The first source produces a pair of photons in the stateand the second produces photons in the state. The signal photons from the first pair are rotated to the state |+ using a half wave plate (HWP) and both signal photons are then fused using a polarizing beam splitter (PBS). The polarizations of the signal photons are then rotated using HWPs to form the three-qubit linear cluster state, where the first idler photoni1is used as a trigger to verify a fourfold coincidence signifying the generation of the state. The path degree of freedom of the signal photons is then used to expand the resource to a five-qubit linear cluster state using a Sagnac interferometer, as shown in the dashed boxes and explained in the main text. Local complementation operations are then carried out to rotate the linear cluster into the graph state shown inb, as detailed in ref.35. (b) Diagram of the secret sharing scenario. Here the vertices correspond to qubits initialized in the state |+ and edges correspond to controlled-phase gates,CZ=diag(1, 1, 1, −1), applied to the qubits. Figure 1: Experimental setup. ( a ) Setup used to generate the graph state resource for secret sharing. Two photonic crystal fibre (PCF) sources are pumped using a Ti:Sapphire laser producing picosecond pulses at 724 nm. The first source produces a pair of photons in the state and the second produces photons in the state . The signal photons from the first pair are rotated to the state |+ using a half wave plate (HWP) and both signal photons are then fused using a polarizing beam splitter (PBS). The polarizations of the signal photons are then rotated using HWPs to form the three-qubit linear cluster state , where the first idler photon i 1 is used as a trigger to verify a fourfold coincidence signifying the generation of the state. The path degree of freedom of the signal photons is then used to expand the resource to a five-qubit linear cluster state using a Sagnac interferometer, as shown in the dashed boxes and explained in the main text. Local complementation operations are then carried out to rotate the linear cluster into the graph state shown in b , as detailed in ref. 35 . ( b ) Diagram of the secret sharing scenario. Here the vertices correspond to qubits initialized in the state |+ and edges correspond to controlled-phase gates, C Z =diag(1, 1, 1, −1), applied to the qubits. Full size image Additional qubits are then added to the linear graph state by expanding the signal photons into two paths in displaced Sagnac interferometers, with the extra degree of freedom associated with the path of the photon corresponding to a qubit in each interferometer. The beamsplitters used in the interferometers are hybrids, with half of their surface a PBS and the other half a 50:50 beamsplitter (BS). The signal photons are input through the PBSs, so that their paths are correlated with their polarizations and the graph state is extended by a qubit at each end, creating a five-qubit linear graph. This is equivalent to the resource state shown in Fig. 1b up to local complementation operations [37] , which are carried out using additional waveplates and a relabelling of the interferometer paths to the Pauli X basis (see Methods). The five-qubit graph state generated in the experiment and shown in Fig. 1b is given explicitly by where the eigenstates of the Pauli Y operator are . To measure the path qubit in the Pauli X basis, one path or the other is blocked inside the interferometer. To measure in the Y or Z basis, the paths are allowed to recombine at the BS surface with different relative phases. The polarization qubits are then measured using quarter-wave plate–HWP–PBS chains, followed by silicon avalanche photodiode detectors, which enable any Pauli basis measurement to be performed [40] . Before demonstrating secret sharing with the graph state, we first checked for the presence of entanglement using an entanglement witness [41] . In this case, it is possible to detect genuine multipartite entanglement in a linear cluster state using the correlations from only two local measurement bases. Since the five-qubit graph state is locally equivalent to a five-qubit linear cluster state, by making corresponding changes to the reference frames of the measurements we obtain the relevant witness (see Methods). The measurements are X 0 X 1 X 2 X 3 X 4 and Y 0 Z 1 Y 2 Y 3 Z 4 , which lead to a witness value of =−0.15±0.03. The error is calculated using a Monte Carlo method with Poissonian noise on the count statistics [40] . The negative expectation value of the witness reveals the presence of genuine multipartite entanglement and confirms that all qubits are involved in the generation of the graph state. We also obtain the fidelity of the experimental graph state with respect to the ideal case using seventeen measurement bases (see Methods) and find a fidelity of F =0.70±0.01. Having characterized the resource state, we move onto testing its performance in carrying out secret sharing protocols. We consider qubit 0 to belong to the dealer, and qubits 1, 2, 3 and 4 to players 1, 2, 3 and 4 respectively. It can be seen from equation (1) that the graph state is a maximally entangled state between the dealer and the players. Thus, its use for secret sharing can be thought of as analogous to the way a maximally entangled state is used for two player communication. When using it to share a classical secret, a random key can be established between the dealer and authorized sets of players, similar to entanglement-based quantum key distribution (QKD) [38] . On the other hand, when using it to share a quantum secret it can be thought of as the entangled resource for teleporting a secret state from the dealer to the players. In both cases, the shape of the graph state imposes restrictions on which sets of players can access the secret, giving the overall access structure for the secret sharing. The more complex structure of our graph state resource compared to previously used GHZ states [42] , [43] , [44] , [45] , [46] , for example, means that it can achieve more general access structures. Indeed, all access structures are possible using generalized graph states [47] . Classical secret sharing In the CQ protocol, the graph state in equation (1) is used to establish a random bit string, or ‘key’, which can be known only by the dealer and an authorized set of players [14] , [18] . In this sense, it is similar to a secret key generation protocol: once the key is established, it can be used to securely communicate secret classical information between the dealer and the authorised set of players, even in the presence of eavesdroppers (making it an improvement on the Shamir–Blakely schemes [16] , [17] , which require trusted channels). We will see later that it also can be used as a subprotocol for secure quantum secret sharing (SQQ). As in entanglement-based QKD, the players both measure in randomly chosen complementary bases, the correlations are then checked, and if sufficiently high the shared key can be trusted. The dealer starts by measuring their qubit either in the Pauli Y or Z basis, chosen at random. Thus, the dealer’s measurement projects the players’ state into one of four states , where j =( Z , Y ) represents the dealer’s basis choice and i =(0,1) the dealer’s measurement result. The four possible states can easily be calculated from equation (1). The dealer’s result is used as the secret key and the task of the players is to make measurements to discriminate the four states and find i . They cannot do this perfectly without knowledge of the basis choice j , so they make choices based on a guess j ′ for the basis used by the dealer. As in standard QKD, after the players measure their qubit, the basis choice j is announced by the dealer. If the players’ measurements were chosen differently, that is, j ′≠ j , the results are discarded. A ‘sifted’ key is built up using the cases where the bases of the dealer and the players coincide. For a given basis choice j of the dealer, a set of players is ‘unauthorized’ if there is no measurement they can make to find i , and a set of players is ‘authorized’ if they are able to perfectly find i using particular measurements. Further details of this protocol and its proof of security can be found in refs 16 , 36 . To check whether a set of players, B , that use the five-qubit graph state generated in our experiment can access the secret, it is necessary to look at their reduced states given the dealer’s result and basis choice. To quantify how well a set of players can access the dealer’s results, we use the accessible information [38] , , where S ( ρ ) is the von Neuman entropy of state ρ and and p i , j is the probability the dealer obtains result i when measuring basis j . This allows us to quantify the maximum possible information that the players in set B can obtain about the dealer’s results for a given basis choice j . When χ j is zero, there is no information that the players can obtain about the dealer’s result, no matter which measurements they make. Indeed, it can be shown (see Methods) that using the state in equation (1) a single player cannot obtain any information about the dealer’s result. That is, their reduced density matrix is independent of the dealer's result i , for both bases j . In Fig. 2 , we have measured the reduced density matrices for each player (for each of the dealer’s results) from our graph state to obtain the accessible information χ . One can see from Fig. 2a,b that the accessible information about the dealer’s results are very close to zero for both the Z and Y bases, confirming that individual players have almost zero information about the dealer’s results. 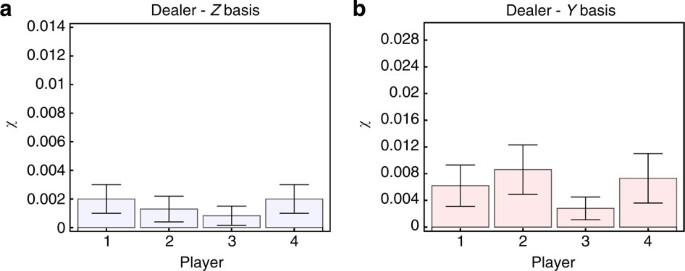Figure 2: Accessible information for single players in classical secret sharing using the graph state. (a) Accessible informationχfor single players when the dealer measures inZ. (b) Accessible informationχfor single players when the dealer measures inY. In both panels it is clear that when acting alone the players have almost zero information about the state the dealer has prepared. Error bars are calculated using a Monte Carlo method with Poissonian noise on the count statistics40. Figure 2: Accessible information for single players in classical secret sharing using the graph state. ( a ) Accessible information χ for single players when the dealer measures in Z . ( b ) Accessible information χ for single players when the dealer measures in Y . In both panels it is clear that when acting alone the players have almost zero information about the state the dealer has prepared. Error bars are calculated using a Monte Carlo method with Poissonian noise on the count statistics [40] . Full size image We have also checked the density matrices of the individual players. Before the dealer makes a measurement, the fidelities of the single-player reduced density matrices with respect to a maximally mixed state I /2 are F =0.961±0.005, 0.996±0.002, 0.998±0.001 and 0.996±0.002 for players 1, 2, 3 and 4, respectively. Once the dealer makes a measurement, the four different states for each player (two for when the dealer measures in the Z basis and two for the Y basis) remain close to the maximally mixed state, leading to the low values of measured accessible information shown in Fig. 2 . When pairs of players try to work together to recover the secret key, there are two cases, with the amount of information accessible different if the pair are adjacent: {1, 3}, {1, 4}, {2, 3} and {2, 4} or diagonally opposite: {1, 2} and {3, 4}. It can easily be shown that a given pair of adjacent players cannot obtain any information about the dealer’s result from the state in equation (1) (see Methods). One can see from Fig. 3a,b that the accessible information about the dealer’s results are very close to zero for both the Z and Y bases, confirming that adjacent pairs of players have almost zero information about the dealer’s results. On the other hand, when a pair of players are at opposite corners, it can be shown using equations (1) and (8) that when the dealer measures in the Z basis they obtain no information, but when they measure in the Y basis they obtain full information. For example, the pair {3, 4} could do this by measuring their qubits in the bases Z 3 and Y 4 . If the results are correlated, the dealer’s result would be 1, if they are anticorrelated it would be 0. Similar conclusions can be found for the pair {1, 2}. In Fig. 3c,d , one can see that the measured accessible information about the dealer’s results is very close to zero for the Z basis, but significantly larger for the Y basis, confirming that opposite pairs of players can access information about the dealer's results. 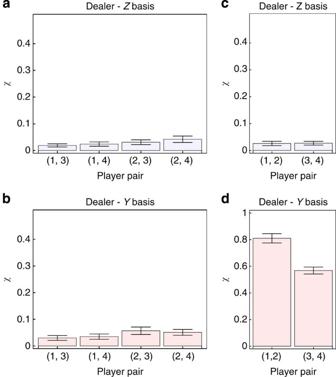Figure 3: Accessible information for two players in classical secret sharing using the graph state. a(c) Accessible informationχfor pairs of adjacent (opposite) players when the dealer measures inZ.b(d) Accessible informationχfor pairs of adjacent (opposite) players when the dealer measures inY. From the panels, it is clear that only opposite players have some information about the state the dealer has prepared when the dealer measures in theYbasis. Error bars are calculated using a Monte Carlo method with Poissonian noise on the count statistics. Figure 3: Accessible information for two players in classical secret sharing using the graph state. a ( c ) Accessible information χ for pairs of adjacent (opposite) players when the dealer measures in Z . b ( d ) Accessible information χ for pairs of adjacent (opposite) players when the dealer measures in Y . From the panels, it is clear that only opposite players have some information about the state the dealer has prepared when the dealer measures in the Y basis. Error bars are calculated using a Monte Carlo method with Poissonian noise on the count statistics. Full size image Finally, if three players work together, then it can be shown that in the ideal case they can access the dealer’s measurement result perfectly for both the Z and Y bases. For example, if the dealer measures in the Y basis, the triplet of players {1, 2, 4} can retrieve the result by measuring their qubits in the bases Z 2 and X 4 , with the result of the dealer’s outcome obtained from the measurement of designated player 1 in the Y basis after feedforward operations are applied (where s i =(0,1) represents the outcome of the measurement of qubit i ). This scenario also holds for the Z basis of the dealer. The above results can easily be checked by inspection of equation (1). The same retrieval process of the dealer’s measurement result holds for any triplet of players by symmetry. The correlations within the graph state can therefore be used to establish a shared random key between the dealer and any set of three players. In Fig. 4 , we show the measured quantum bit error rates (QBERs) for generating a shared random key for the four possible triplets of players: {1, 2, 3}, {1, 2, 4}, {2, 3, 4} and {1, 3, 4}. The result of the dealer is obtained from the measurement of a designated player’s qubit. 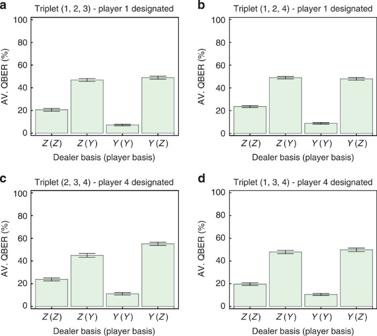Figure 4: QBERs for three players in classical secret sharing using the graph state. (a–d) Average QBER for the bit retrieved by the three player triplets when working together, with the bit retrieved by a designated player. For the designated player, the measured bit outcomes are correlated in the same bases as the dealer (ideally zero QBER) and uncorrelated in the opposite bases (ideally 50% QBER). Error bars are calculated using a Monte Carlo method with Poissonian noise on the count statistics. Figure 4: QBERs for three players in classical secret sharing using the graph state. ( a – d ) Average QBER for the bit retrieved by the three player triplets when working together, with the bit retrieved by a designated player. For the designated player, the measured bit outcomes are correlated in the same bases as the dealer (ideally zero QBER) and uncorrelated in the opposite bases (ideally 50% QBER). Error bars are calculated using a Monte Carlo method with Poissonian noise on the count statistics. Full size image We can also check what happens to the accessible information from the QBER values. Once the measurement basis is chosen by the players and the dealer, a non-zero QBER with value p represents the action of the superoperator . It is not difficult to see that for p =50% the accessible information will be zero, irrespective of . In Fig. 4 , one can see that the QBERs are low when the dealer and designated player measure in the same basis and close to 50% when they use a different basis—corresponding to completely uncorrelated results with no accessible information for the players. By taking the QBERs from both the Z and Y bases, when the dealer and designated player measure in the same bases, we almost reach the 11% bound needed to establish a secure random key [5] . We obtain 14±2, 16±2, 18±2 and 15±2% for the triplets {1, 2, 3}, {1, 2, 4}, {2, 3, 4} and {1, 3, 4}, respectively. Although these QBERs are just above the secure bound, the results demonstrate a first implementation of QKD with the access structure of the graph state. Note also that in our experiment, the players do not receive separate photons as we are making use of hyperentanglement [21] , [22] , [23] . This means that qubits 1 and 2 are embodied by one photon, and qubits 3 and 4 by another. Thus, one photon would belong to players 1 and 2, while the other to players 3 and 4. For a pair of players that share a single photon, one can split up the access sets into their original form by allowing one player to control the measurement setting and readout of the path qubit, and the other to control the setting and readout of the polarization qubit. In this way, the hyperentangled state can in principle be shared out to four players at spatially separate locations. To do this, the dealer would send one of the photons to the first player of a pair, who measures the path qubit using a quantum non-demolition measurement [48] and then forwards the photon to the second player at a separate location to measure the polarization qubit. To check for any eavesdropping by the first player, the dealer could at random intervals send a decoy qubit (in the polarization basis) to the players of a pair and together with the second player check for eavesdropping using standard BB84 methods [5] . From a practical point-of-view, it may therefore be more straightforward for each player to receive a separate photon (each encoding one qubit of the graph state), although this would require modifying the present experimental setup. In summary, using the graph state generated in our setup to share classical information via quantum channels (CQ), we have demonstrated a secret sharing scheme where a secret is distributed across four players such that any three can access the secret and any single player obtains no information. This is known as a ramp scheme with parameters (3, 1, 4). Here a ramp scheme ( k , k ′, n ) enables the parameterizing of any secret sharing scheme over n players such that any set of k or more players have perfect access to the secret and any set of k ′ or fewer players have no access to the secret. If k ′= k −1, then the scheme is called a ( k , n ) threshold scheme. Quantum secret sharing We now show how our generated graph state can also be used to implement a (3, 1, 4) ramp scheme for sharing a quantum secret using the method described in ref. 16 . We then show how this ramp scheme can be upgraded to a (3, 4) threshold scheme via hybrid quantum secret sharing (using both classical and quantum secret sharing) [49] , [50] . That is, any three players can access the quantum secret, but any fewer cannot. This is known to be impossible using a qubit pure quantum secret sharing protocol alone, that is, without some classical mixing [18] , [38] . In the QQ protocol, a quantum state (the quantum secret) is encoded by the dealer onto the following four-qubit state shared by the players where | φ 1234 =(1/2)(|++00+|++11+|−−01+|−−10) 1234 is a square graph state and | φ ′ 1234 = Z 1 Z 2 Z 3 Z 4 | φ 1234 . The dealer achieves this encoding by teleporting in their secret state via a Bell measurement of the joint state of and qubit 0 of the graph given in equation (1) [36] , [49] . Alternatively, the dealer can directly prepare qubit 0 of the graph in the secret state and measure it in the X basis with the feedforward operation applied. In our experiment, we implement this latter more compact approach for encoding the secret. The task of a set of players is then to access the secret quantum information. To quantify the amount of information that can be accessed by a set of players B in this quantum version of secret sharing, we use the quantum mutual information of the reduced state shared by the dealer and the set of players [51] , ρ 0, B , which is given by I ( ρ 0, B )= S ( ρ 0 )+ S ( ρ B )− S ( ρ 0, B ), where ρ 0 and ρ B are the reduced states of the dealer and players, respectively. If I ( ρ 0, B ) is zero, the players obtain no information about the quantum secret. For any single player, it can be shown that the encoding in equation (2) leads to a reduced density matrix that is maximally mixed, independent of the secret input qubit. In Fig. 5 , we have used quantum process tomography and treated the communication between the dealer and each player as a quantum channel for the secret qubit to be transferred over. Here four probe states are used for the dealer's secret qubit, |0, |1, |+ and |+ y , which enable the reconstruction of the final Bloch sphere obtained by each of the players. One can see from Fig. 5 that all of the dealer’s secret qubit states are transferred to states close to the maximally mixed state for the players. Furthermore, the measured mutual information between the dealer and each player, given in the caption, is consistently close to zero. Thus, a single player acting alone cannot obtain any information about the shared quantum secret. 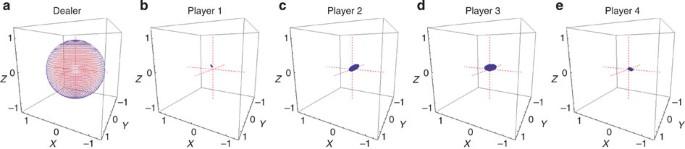Figure 5: Accessible information for single players in quantum secret sharing using the graph state. Single-qubit Bloch spheres for individual players. Here each Bloch sphere represents the output qubit states for an arbitrary state encoded by the dealer. (a) Original Bloch sphere of states encoded by the dealer. (b) Player 1 Bloch sphere. (c) Player 2 Bloch sphere. (d) Player 3 Bloch sphere. (e) Player 4 Bloch sphere. One can see the Bloch spheres all correspond to an almost completely mixed stateI/2 for the dealer’s input states. The corresponding mutual information shared between the dealer and players 1, 2, 3 and 4 isI=0.005±0.001, 0.009±0.002, 0.013±0.003 and 0.009±0.003. The process fidelity of the channel describing the mapping of the dealer’s states to the players states is given by60, whereχidis an ideal maximally mixed channel andχexpis the experimentally reconstructed one. From this definition, we obtain process fidelities of 0.989±0.002, 0.973±0.043, 0.980±0.005 and 0.975±0.056 for players 1, 2, 3 and 4, respectively. Thus, in the one-player case, the players have almost no information about the state the dealer has shared using the graph state. Error bars are calculated using a Monte Carlo method with Poissonian noise on the count statistics. Figure 5: Accessible information for single players in quantum secret sharing using the graph state. Single-qubit Bloch spheres for individual players. Here each Bloch sphere represents the output qubit states for an arbitrary state encoded by the dealer. ( a ) Original Bloch sphere of states encoded by the dealer. ( b ) Player 1 Bloch sphere. ( c ) Player 2 Bloch sphere. ( d ) Player 3 Bloch sphere. ( e ) Player 4 Bloch sphere. One can see the Bloch spheres all correspond to an almost completely mixed state I /2 for the dealer’s input states. The corresponding mutual information shared between the dealer and players 1, 2, 3 and 4 is I =0.005±0.001, 0.009±0.002, 0.013±0.003 and 0.009±0.003. The process fidelity of the channel describing the mapping of the dealer’s states to the players states is given by [60] , where χ id is an ideal maximally mixed channel and χ exp is the experimentally reconstructed one. From this definition, we obtain process fidelities of 0.989±0.002, 0.973±0.043, 0.980±0.005 and 0.975±0.056 for players 1, 2, 3 and 4, respectively. Thus, in the one-player case, the players have almost no information about the state the dealer has shared using the graph state. Error bars are calculated using a Monte Carlo method with Poissonian noise on the count statistics. Full size image For pairs of players, the situation changes with regards to the amount of accessible information. When the players are adjacent, they obtain no information in the Z – Y plane of the secret qubit’s Bloch sphere, but they can obtain information in the Z – X and X – Y planes (see Methods). In Fig. 6a–c , we show the experimental results from the player pair {1, 4}. Here we plot the fidelity between the players’ two-qubit state and fixed states as the dealer varies the angles in the respective planes of the Bloch sphere for their secret qubit. This fidelity gives us an indication of how the state of the pair changes based on the dealer’s input state. In Fig. 6a , the fixed state is I /4 for the Z – Y plane. In Fig. 6b,c , the fixed states are the orthogonal states and for both the Z – X and X – Y planes. Essentially, the oscillations between the fixed orthogonal states show that some information about the dealer’s qubit remains in the joint state of the two players and depends on the plane in which the qubit is encoded into. We quantify the amount of secret information in the adjacent pair of player’s qubits using the mutual information of the state shared by the dealer and the pair, measuring a value of I =0.29±0.02, obtained from a three-qubit state tomography. This shows that some of the secret quantum information is shared between the dealer and adjacent pairs of players. 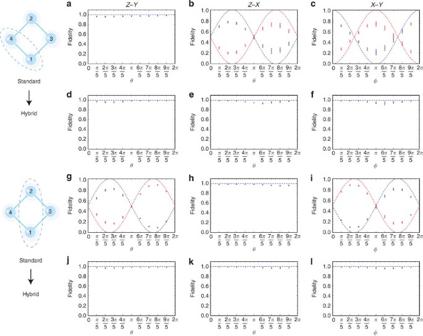Figure 6: Accessible information for two players in quantum secret sharing using the graph state. The fidelities with respect to fixed reference states for the two-qubit states shared by two players as the dealer encodes qubit states into the graph along three orthogonal Bloch sphere planesZ–Y,Z–XandX–Y(parameterized by the canonical anglesθandφ). (a–f) Fidelities for adjacent players (1 and 4), as shown in the illustrations on the left hand side, with panelsa–cshowing the standard encoding scheme, where the mutual information between the dealer and the pair of players isI=0.29±0.02.d–fshow the hybrid encoding scheme used to remove information in all three planes.g–l, fidelities for opposite players (1 and 2), as shown in the illustrations on the left hand side, witha–cshowing the standard encoding scheme, where the mutual information between the dealer and the pair of players isI=0.62±0.02 andd–fshowing the hybrid encoding scheme. The fixed reference states in the panels are as follows: In (a,d–f), the fixed state isI/4. Inb,c, the fixed states are the orthogonal states(red) and(blue). Inh,j–l, the fixed state is. Ing,i, the fixed states are the orthogonal states(red) and(blue). The oscillations between the fixed orthogonal states show that some information about the dealer’s qubit remains in the joint state of two players—depending on the plane the qubit is encoded into and quantified by the mutual information valuesI. However, when the dealer applies the hybrid encoding, the information is almost completely removed as shown by the fidelities remaining constant over the angles of the planes. Error bars are calculated using a Monte Carlo method with Poissonian noise on the count statistics. Figure 6: Accessible information for two players in quantum secret sharing using the graph state. The fidelities with respect to fixed reference states for the two-qubit states shared by two players as the dealer encodes qubit states into the graph along three orthogonal Bloch sphere planes Z – Y , Z – X and X – Y (parameterized by the canonical angles θ and φ ). ( a – f ) Fidelities for adjacent players (1 and 4), as shown in the illustrations on the left hand side, with panels a – c showing the standard encoding scheme, where the mutual information between the dealer and the pair of players is I =0.29±0.02. d – f show the hybrid encoding scheme used to remove information in all three planes. g – l , fidelities for opposite players (1 and 2), as shown in the illustrations on the left hand side, with a – c showing the standard encoding scheme, where the mutual information between the dealer and the pair of players is I =0.62±0.02 and d – f showing the hybrid encoding scheme. The fixed reference states in the panels are as follows: In ( a , d – f ), the fixed state is I /4. In b , c , the fixed states are the orthogonal states (red) and (blue). In h,j – l , the fixed state is . In g,i , the fixed states are the orthogonal states (red) and (blue). The oscillations between the fixed orthogonal states show that some information about the dealer’s qubit remains in the joint state of two players—depending on the plane the qubit is encoded into and quantified by the mutual information values I . However, when the dealer applies the hybrid encoding, the information is almost completely removed as shown by the fidelities remaining constant over the angles of the planes. Error bars are calculated using a Monte Carlo method with Poissonian noise on the count statistics. Full size image On the other hand, when the players are opposite, they obtain no information in the Z – X plane, but can extract information in the Z – Y and X – Y planes. In Fig. 6g–i , we show the experimental results from the player pair {1, 2}. In Fig. 6h , the fixed state is for the Z – X plane, while in Fig. 6g,i , the fixed states are the orthogonal states and for both the Z – Y and X – Y planes. Again, the oscillations between the fixed orthogonal states show that some information about the dealer’s qubit remains in the joint state of two players. In this case, the mutual information of the state shared by the dealer and the pair is measured to be I =0.62±0.02, obtained from three-qubit state tomography. To elevate this secret sharing QQ scenario to a threshold scheme, that is, one where no two players can obtain any quantum information, we use a hybrid protocol [49] , [50] . In this class of protocols, any ( k , k ′, n ) ramp scheme can be elevated to a ( k , n ) threshold scheme, and in fact all intermediate ramp schemes ( k , k ′′, n ) for any k ′ ≤ k ′′ ≤ k −1 can be achieved. In our case, we can elevate the (3, 1, 4) ramp scheme to a (3, 4) threshold scheme. The hybrid scheme uses, in addition to the QQ ramp scheme (already described and characterized), a quantum one-time pad and classical secret sharing. That is, before the encoding, the dealer applies a randomly chosen Pauli operation so that the state encoded is , where x , z are randomly chosen bits by the dealer. This state is then encoded and distributed, and the classical information x , z is shared using classical secret sharing with ramp scheme parameters ( k , k ′′, n ). Without the classical information no players will be able to retrieve , but with the classical information, any k can still access the information perfectly. In the present case, if the classical information is distributed using a classical (3, 4) secret sharing scheme, no two players can know its value and therefore they will not be able to retrieve . We check the performance of the hybrid protocol experimentally by applying randomly the operators I , X , Z and XZ to the dealer’s qubit and measuring the resulting state of the pairs of players. In Fig. 6d–f , we show the fidelity of the adjacent player’s shared state with respect to the fixed state I /4 and in Fig. 6j–l we show the fidelity of the opposite player’s shared state with respect to the fixed state . One can see that when the dealer applies the hybrid encoding protocol, any shared information is almost completely removed from the state corresponding to pairs of players, as shown by the fidelities remaining constant over the angles of the planes. On the other hand, for any set of three players the encoding in equation (2) allows them to access the quantum secret perfectly. For example, if players 2 and 4 measure in Z 2 and X 4 , respectively, the graph state is projected to one where the secret quantum state resides on the qubit of player 1, up to a byproduct operation . The same holds for any three players by symmetry. Thus, for the QQ protocol, all sets of three players can access the secret. When the hybrid protocol is used to remove quantum information from pairs of players, since the classical information of the one-time pad will be known by any set of three players it can easily be undone, allowing any three players to obtain the secret quantum information. In Fig. 7 , we show the results from our generated graph state when the set of players {1, 2, 4} and {2, 3, 4} work to uncover the secret qubit shared by the dealer. Here the designated player who retrieves the secret qubit is player 1 in Fig. 7a and player 4 in Fig. 7b . We again treat the communication from the dealer to the designated player as a quantum channel and carry out quantum process tomography. One can see that in both sets of three players, the secret quantum information is retrieved, although with some deformation of the Bloch sphere caused by the non-ideal graph state used in our experiment. However, the fidelity for an arbitrary qubit shared between the dealer and the set of players {1, 2, 4} averaged over the Bloch sphere remains high with (qubit retrieved by player 1). For the qubit shared between the dealer and the set of players {2, 3, 4}, we have (qubit retrieved by player 4). 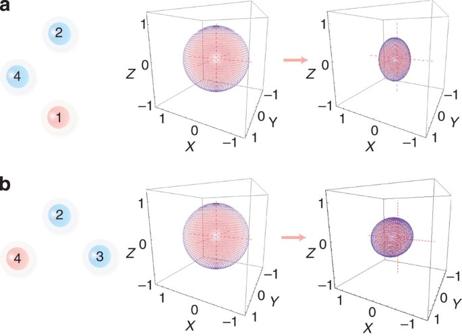Figure 7: Fidelity of recovered quantum secret for three players in quantum secret sharing using the graph state. (a) Bloch sphere of an arbitrary qubit shared by the dealer to players 1, 2 and 4, with the secret residing on the qubit of player 1, as shown in the illustrations on the left hand side with player 1 in red. The average fidelity for a shared qubit is. (b) Bloch sphere for players 2, 3 and 4, with the secret residing on the qubit of player 4, as shown in the illustrations on the left hand side with player 4 in red. The average fidelity for a shared qubit in this case is. In both, the spheres are slightly squashed due to the non-ideal graph state resource used in the experiment. Error bars are calculated using a Monte Carlo method with Poissonian noise on the count statistics. Figure 7: Fidelity of recovered quantum secret for three players in quantum secret sharing using the graph state. ( a ) Bloch sphere of an arbitrary qubit shared by the dealer to players 1, 2 and 4, with the secret residing on the qubit of player 1, as shown in the illustrations on the left hand side with player 1 in red. The average fidelity for a shared qubit is . ( b ) Bloch sphere for players 2, 3 and 4, with the secret residing on the qubit of player 4, as shown in the illustrations on the left hand side with player 4 in red. The average fidelity for a shared qubit in this case is . In both, the spheres are slightly squashed due to the non-ideal graph state resource used in the experiment. Error bars are calculated using a Monte Carlo method with Poissonian noise on the count statistics. Full size image Secure quantum secret sharing Finally, we introduce and demonstrate a new protocol for sharing a quantum secret over untrusted channels between the dealer and the players, which we denote by SQQ (for secure QQ). This is performed here for a (3, 4) threshold scheme, its extension to general access structures is presented in ref. 45 . The QQ protocol (and its hybrid version) detailed previously work as long as the state used for encoding is the same as (or close to) that given in equation (1). However, if the channel from the dealer to the players is noisy or untrusted, this may not be the case. Thus, without knowing the initial secret that was sent, an authorized set of players cannot know if they received it correctly or not. The SQQ protocol rectifies this problem by verifying that the state used is indeed that in equation (1), or close to it. Here CQ measurements are used as a subprotocol to test the resource state (in a similar way to how a GHZ state can be tested using the verification protocol recently presented in ref. 50 ). The protocol works as follows: after generating and distributing the graph state, the dealer decides either to test it, or to use it for quantum secret sharing, with probability 1- s and s , respectively. Here s acts as a security parameter. The dealer announces the choice about whether to test or use it publicly, and the dealer and players carry out their part of the test or the secret sharing scheme, respectively. The test is essentially an adapted version of the CQ protocol, which by checking the correlations of the graph state verifies it is close to the one desired. In the test, the dealer measures in either X , Y or Z , or does not make any measurement, all with equal probability. They then announce their choice and the results publicly. A set of players B who are checking the state then perform measurements depending on the dealer's measurement choice. The measurements used by the sets of three players are explicitly detailed below, along with a description of how the level of security is quantified. It can be shown (see Methods) that if a given resource state ρ shared between the dealer and players is used for quantum secret sharing and the qubit state ω retrieved by an authorized set of players has fidelity f = ψ | ω | ψ with respect to the secret state , then the probability P that the resource state ρ passes the CQ test is related to the fidelity by In other words, a resource state which passes the test with high probability will give a high fidelity when used for secret sharing. Furthermore, if we let C f be the event that the protocol has not aborted and that the state ρ was used for QQ, then the probability P ( C f ) of this event occurring satisfies (see Methods). Thus, if the test is passed in the cases when the dealer announces they should test, then the players can be confident that when the dealer announces they should instead use the state, the secret quantum information retrieved will be of high fidelity. As an example of this protocol using our experimental graph state, we consider the set of players {1, 2, 3}. The same holds for all sets by symmetry. The measurements for the test correspond to randomly measuring one of the following operators Z 0 Z 1 Z 2 X 3 , Y 0 Y 1 Z 2 I 3 , Y 0 Z 1 Y 2 I 3 , X 0 X 1 I 2 X 3 , X 0 I 1 X 2 X 3 , I 0 X 1 X 2 I 3 or Z 0 Y 1 Y 2 X 3 (see Methods). The test is passed if the measurement results for these operators are +1, +1, +1, −1, −1, +1 and −1, respectively. Using the measured expectation values for these operator settings, in Fig. 8a , we show the probability that our experimental state passes the test and in Fig. 8b we show the corresponding lower bounds on the fidelity, which are consistent with the fidelities measured previously in Fig. 7 . Thus, using the verified protocol, we find that the probability of the experimental resource state passing the test is fully consistent with the previously measured fidelity of the retrieved secret qubit states obtained by the three players. 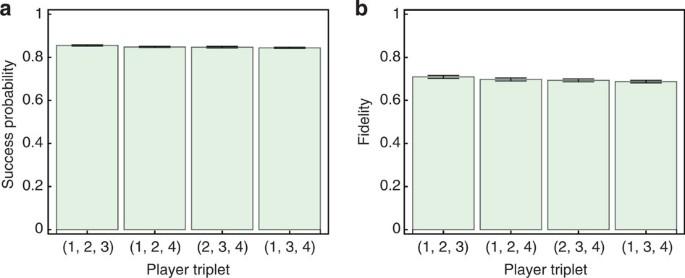Figure 8: Verified quantum secret sharing protocol. (a) Expected success probabilities for the protocol being carried out between the dealer and different sets (triplets) of three players. The success of the verified protocol (see text for details) allows the dealer to verify the access structure of the graph resource and carry out verified quantum secret sharing. (b) Lower bound on the fidelity of the state shared by the players with respect to the ideal graph state. Error bars are calculated using a Monte Carlo method with Poissonian noise on the count statistics. Figure 8: Verified quantum secret sharing protocol. ( a ) Expected success probabilities for the protocol being carried out between the dealer and different sets (triplets) of three players. The success of the verified protocol (see text for details) allows the dealer to verify the access structure of the graph resource and carry out verified quantum secret sharing. ( b ) Lower bound on the fidelity of the state shared by the players with respect to the ideal graph state. Error bars are calculated using a Monte Carlo method with Poissonian noise on the count statistics. Full size image While previous experiments on quantum secret sharing focused on sharing classical secrets [42] , [43] , [44] , [45] , [46] , with some work regarding the sharing of quantum secrets amongst three players [53] , [54] , [55] , [56] , [57] , our work goes beyond these studies in two crucial aspects. First, the secret sharing is performed using graph states, which are of great importance for the integration of secret sharing with a wide range of quantum networking protocols via the measurement-based paradigm [28] . In our experiment, we demonstrated the use of graph states for both classical (CQ) and quantum (QQ) secret sharing. We used a photonic setup to generate a five-qubit graph state and carried out the encoding, sharing and retrieval of classical and quantum secrets. In the CQ protocol we demonstrated the ability of the graph to share a classical random key, which can be used to securely share classical secrets, with an access structure of a (3, 1, 4) ramp scheme. Here the secret is shared between four players, such that any three can perfectly access the secret, yet no single player obtains any information at all. The QQ protocol achieves the same access structure for a quantum secret. However, the second crucial aspect of our work that puts it beyond previous studies is that with the integration of several different cryptographic sub-protocols (one classical and two quantum), the (3, 1, 4) access structure for the QQ protocol is elevated to a (3, 4) threshold scheme, that is, any three players can access the quantum secret, but fewer have no information. This hybrid QQ protocol is a combination of classical secret sharing and the QQ protocol, which allows us to achieve an access structure known to be impossible with QQ alone. We then introduced and demonstrated a new protocol for sharing a quantum secret over untrusted channels, which we call SQQ. Taken together with the hybrid QQ protocol, this highlights the power of integrating tasks via the hybridization of classical and quantum protocols using the graph state approach, and enables us to achieve protocol parameters and security not possible with any single protocol. In terms of a real world use of graph states for quantum secret sharing, practical security considerations will need to be taken into account, such as imperfections in the generation of the resource, as well as noise and loss effects during the transfer of the photons over communication networks. All these factors will reduce the security of the scheme and this is an important topic for future studies of graph state quantum secret sharing. As more sophisticated ways of using graph states emerge, combining and demonstrating different sub-protocols in the way we have done here will become increasingly more relevant. The facility and flexibility of graph states for different quantum information processing tasks clearly propels them forward as a technology with great potential for future quantum networks. Experimental setup The PCF sources used in the experiment are similar to those described in refs 56 , 57 . When pumped by picosecond pulses from a Ti:Sapphire laser at 724 nm on the slow birefringent axis of the PCF, spontaneous four-wave mixing produces signal–idler photon pairs at 625 and 860 nm, polarized on the fast axis of the fibre. The cross-polarized phase-matching scheme takes advantage of a turning point in the signal wavelength where it is locally independent of the pump wavelength, which has the effect of avoiding correlations between the signal and idler’s spectra. This allows quantum interference to take place between photons from separate sources without the need for tight spectral filtering, which would reduce the collection efficiency. To produce signal–idler pairs in a polarization Bell state, the PCF is set up in a Sagnac loop around a PBS and pumped in both directions. The axes of the fibre are twisted so that in the clockwise direction around the loop, the photon pairs polarized on the fast axis emerge horizontally polarized, while for the counter-clockwise direction, photon pairs emerge vertically polarized. When the two directions are recombined at the PBS, all the photon pairs exit through the same output, so that the state of a single pair in this beam is in a superposition , where the phase θ between the two directions can be tuned to zero using a birefringent compensator placed in the pump beam before the loop. The other PCF source is pumped in a single direction so as to produce pairs without polarization entanglement. The idler is detected as a heralding photon, while the signal photon is rotated to diagonal polarization . This is then overlapped at the fusion PBS with the signal photon from the other source and we postselect events for the cases where one signal emerges from each PBS output. This implies that the two signal photons have the same polarization, or are in an even parity state, so that they have either both been transmitted or both been reflected at the PBS. The conditioned state is a three-photon GHZ state , which is converted to a linear graph state by waveplate rotations applied to the signal modes. Each signal photon is then launched into a displaced Sagnac interferometer. Here they are split at the PBS surface of the hybrid beamsplitters, and we label the transmitted paths the |0 states of the path qubits, and the reflected paths the |1 states. This results in the five-qubit state: which is locally equivalent to a linear graph state and the target resource state, which can be written as: where the eigenstates of the Pauli Y operator are . The required local rotations are implemented by relabelling the transmitted and reflected interferometer paths to |+ and |−, applying HWP rotations to the signal polarizations, and a quarter-wave plate rotation to the idler. Tilted glass plates in each path are used for the relative phase-shifts in the interferometers. To experimentally implement the removal or tracing out of a path qubit (corresponding player does not take part in the secret sharing), the glass plate was removed from one path, so that the two path lengths would differ by more than a coherence length. Hence, the paths are incoherently recombined at the BS surface before going to polarization analysis. This allowed the photon’s polarization to still be detected, but no information was gained about the path. On the other hand, to remove a polarization qubit, the PBS was taken away from the polarization analysis, so that the path information was still detected, but no polarization information was measured. The twofold coincidence rates collected from individual sources were around 9,000 s −1 . Fourfold coincidences where the fusion succeeded, between the three entangled photons and the one herald photon, were ~0.25 s −1 . Generating entanglement relies on the signal photons from separate sources being indistinguishable when they are overlapped at the PBS, otherwise the fusion can only leave an incoherent mix of possibilities [39] . When the relative arrival time of the signal photons was varied, with the measurement bases set appropriately, an anti-dip was seen at zero-delay with visibility ~62%. This indicates there are some distinguishability issues, which will degrade the quality of the state, which mainly result from inhomogeneity along the length of the PCF sources. Resource characterization For the five-qubit graph state, we use the following entanglement witness on qubits 0, 1, 2, 3 and 4 where Õ corresponds to measurements in the O basis with the eigenstates swapped. This is a locally rotated version of the witness given in ref. 39 for a five-qubit linear cluster state and takes into account the required local complementation operations [37] . To obtain the fidelity for the five-qubit graph state, we decompose the fidelity operator into a summation of products of Pauli matrices as Calculating the expectation value of this operator requires 17 unique measurement bases: XXXXX , YXXYZ , YXXZY , ZXXYY , ZXXZZ , XYYYY , XYYZZ , ZYYXX , YYZYZ , XYZZY , YYZXX , YZYYZ , ZZYZY , YZYXX , XZZYY , XZZZZ and ZZZXX . Classical secret sharing To begin, it is useful to rewrite the state the state in equation (1) in an alternative form with the dealer’s qubit in the Z basis, It can be seen by inspection of equations (1) and (8) that the reduced density matrix of any player a is for all basis choices j and results i of the dealer’s measurements. From this it can easily be checked that χ j =0 for all bases j . Hence, no single party can obtain any information. For a pair of players ( a , b ) that are adjacent, one can easily check from equation (1) that , j = Z , Y . Hence, no information can be extracted and χ j =0 for all bases j . For a pair of players ( a , b ) that are opposite it can easily be seen from equation (1) that for j = Y they can access the result by measuring one qubit in Y and the other in Z . Hence, χ Y =1. It can also be shown that for both results i , so that no information can be extracted and χ Z =0. Any triplet of players can access the secret, as discussed in the Results section, which can be seen by inspection of equations (1) and (8). Quantum secret sharing Here we show which players can and which cannot access the secret in the QQ protocol. The first step in the protocol is that the dealer generates and distributes the state in equation (1). We rewrite the state as follows This is used to teleport a secret state to the players. The dealer measures the secret qubit and their part of the state in equation (9) in the Bell basis and announces the results publicly. In the retrieval step, the authorized sets then apply the appropriate correction and the decoding operations. To study the accessibility of the quantum information, we ignore the correction step and assume it is always the good result where no correction is required—if a set of players cannot access the secret for the corrected state, then they cannot access it for the uncorrected state. Similarly, if they can, knowing the results of the dealer’s measurement allows them to do the correction afterwards. Thus, consider the secret teleported to the players, giving the state Note that this state is cyclically symmetric amongst the four players, according to the symmetry of the graph, in this case a square. It can be seen from equation (10) that any single player a has the reduced density matrix ρ a = I /2, thus they cannot access any information. This is quantified by considering the reduced state of equation (9) for ρ 0 a = I /4, so that the mutual information I ( ρ 0 a )=0. For two adjacent players a and b , we have from equation (10) From this we find that they can obtain some information as follows: player a measures in the Z basis (the result of which we denote s a ), and then tells player b the outcome. Player b then performs the correction and we are left with the state on player b as . Thus, in some cases, the full information can be retrieved and in other cases only partially, depending on the secret shared. For example, if the secret state is |± then full information can be retrieved. On the other hand, after teleportation, two opposite players a and b share the state where , , and we take the standard Bloch sphere parameterization of the input qubit α =cos( θ /2) and β = e iφ sin( θ /2). The players can retrieve information as follows: player a measures in the Z basis, obtaining result s a , and player b performs the correction operation . The resulting state is . Thus, in some cases the full information can be retrieved and in other cases only partially, depending on the secret shared. For example, if the secret state is |± y › then full information can be retrieved. For three players, it can easily be seen from the decomposition of equation (9) that if player 2 measures Z 2 and player 4 measures X 4 , the secret can be retrieved on the qubit of player 1 up to feedforward operations . Similar results hold for all sets of three players by symmetry of the graph state. Hybrid quantum secret sharing After the random application of the operators I , X , Z and XZ based on the results of a one-time pad, as well as the QQ encoding teleportation stage, the state of the players is where X L = Z 1 Z 2 X 3 I 4 and Z L = Z 1 Z 2 Z 3 Z 4 . From the arguments in the previous section, players who cannot access the quantum secret in the QQ case cannot access it in this case too. However, players also cannot access anything when they do not know the values x and z . This can be checked by looking at the reduced density matrices mixed over the values of x and z . Thus, any two players not knowing x and z obtain no information, but any three knowing x and z can access the secret state perfectly. Sharing the classical information of x and z via a (3, 4) Shamir–Blakely [16] , [17] classical secret sharing scheme achieves this exactly. Note, we are assuming authenticated classical channels, as in all our schemes. However, to use the Shamir–Blakely [16] , [17] secret sharing scheme one also requires a trusted channel. If one does not trust the classical channels, one could use a CQ scheme to send this information, or indeed the Shamir–Blakely scheme plus multiple standard two party QKD. Secure quantum secret sharing We now present the verified SQQ protocol and its proof in more detail. We exemplify the protocol for our state with accessing set B ={1, 2, 3}. The same steps can be performed by symmetry for all sets of three players. 1 The dealer distributes the players’ qubits of the entangled graph state, that is, the channel state in equation (1). 2 The dealer randomly decides that they will carry out: (a) the protocol or (b) the QQ protocol, with probabilities 1- s and s , respectively, and announces the choice to all players. The protocol defined for an authorized set B ={1, 2, 3}: 1 The dealer chooses randomly which of the seven measurements below should be performed for the test, announcing the choice and results of their part of the measurement (in the case where they are asked to measure I 0 they output the result +1). The minus signs can be interpreted as meaning that the product of outputs should ideally be minus one. 2 To comply, players in B perform their parts of the measurement chosen by the dealer. They then check their correlations by communicating amongst themselves. If the product of outcomes of the dealer and all B is 1 (or −1 according to the sign of the measurement), they give the response ‘pass’, otherwise ‘fail’. 3 If ‘pass’ is returned, proceed to the start of the protocol again, otherwise abort. The QQ protocol defined for the authorised set B ={1, 2, 3}: 1 The dealer measures the quantum secret and their part of the shared channel state in the Bell basis and announces the result. 2 Players B perform the corrections and decoding operation. We now give a proof of the security for the QSS protocol, that is, we prove the fidelity bounds with respect to passing the test. Carrying out the protocol as defined above for players {1, 2, 3} is equivalent to performing a POVM { M pass , M fail }, where M pass is the sum of all the +1 projections for the measurements performed in the , which can easily be seen to give where Γ=(| g 0123 g |+ I 0 Z 1 Z 2 Z 3 | g 0123 g | I 0 Z 1 Z 2 Z 3 ) is the projection onto a space where the QQ protocol works perfectly, and | g 0123 is the graph state of the subgraph of qubits 0, 1, 2 and 3. The probability P of passing the CQ test , given a state ρ , is then given by Consider ρ is now used instead to share a quantum secret | ψ via the QQ protocol. If we denote the fidelity of the decoded state ω , then it follows that f ≥Tr( ρ Γ), since any state in the subspace Γ perfectly transports the secret, so the final fidelity can only be higher than the overlap with this space, giving equation (3). Following the logic in ref. 50 , if we denote C f the event that the certified protocol has not aborted and that the state ρ was used for QQ such that it returns a decoded state with fidelity f with the original secret, then it can be shown that the probability P ( C f ) of this event satisfies This implies that if the test passes, then the fidelity of the output state is high. This relationship is demonstrated in the results section. A generalization of this protocol, with a more detailed and general proof can be found in ref. 45 . How to cite this article: Bell, B. A. et al . Experimental demonstration of graph-state quantum secret sharing. Nat. Commun. 5:5480 doi: 10.1038/ncomms6480 (2014).